Late Cretaceous origin of the rice tribe provides evidence for early diversification in Poaceae Rice and its relatives are a focal point in agricultural and evolutionary science, but a paucity of fossils has obscured their deep-time history. Previously described cuticles with silica bodies (phytoliths) from the Late Cretaceous period (67–65 Ma) of India indicate that, by the latest Cretaceous, the grass family (Poaceae) consisted of members of the modern subclades PACMAD (Panicoideae–Aristidoideae–Chloridoideae–Micrairoideae–Arundinoideae–Danthonioideae) and BEP (Bambusoideae–Ehrhartoideae–Pooideae), including a taxon with proposed affinities to Ehrhartoideae. Here we describe additional fossils and show that, based on phylogenetic analyses that combine molecular genetic data and epidermal and phytolith features across Poaceae, these can be assigned to the rice tribe, Oryzeae, of grass subfamily Ehrhartoideae. The new Oryzeae fossils suggest substantial diversification within Ehrhartoideae by the Late Cretaceous, pushing back the time of origin of Poaceae as a whole. These results, therefore, necessitate a re-evaluation of current models for grass evolution and palaeobiogeography. The critical dependence of humans on rice ( Oryza sativa ) as a crop species has made it a major research focus in both basic and applied plant science [1] , [2] , [3] . Numerous studies have sought to elucidate its domestication history [4] , [5] , [6] , [7] clarify the relationships of species within the genus Oryza and to other genera in the rice tribe [2] , [8] , [9] , [10] , [11] , and track the evolutionary history of the subfamily that rice belongs to, Ehrhartoideae, within the grass family as a whole [12] , [13] , [14] . In these studies, the Ehrhartoideae is reconstructed as consisting of the tribes Oryzeae, Ehrharteae and Phyllorachidae [15] . The subfamily is commonly found to be nested within a monophyletic group consisting of the Bambusoideae, Ehrhartoideae and the Pooideae (the BEP clade) [13] , [16] , [17] ; alternatively, the Bambusoideae, Ehrhartoideae and the Pooideae clades form a paraphyletic grade with reference to the PACMAD (Panicoideae–Aristidoideae–Chloridoideae–Micrairoideae–Arundinoideae–Danthonioideae) clade, with Pooideae as the sister taxon to the PACMADs [18] , [19] . Recent molecular clock estimates calibrated by selected grass fossils indicate that the Ehrhartoideae arose after the K–Pg (Cretaceous–Paleogene) boundary, by the Early Eocene ( ∼ 53 Ma) [17] , that the Oryzeae diverged from the Ehrharteae by the Late Eocene–Early Oligocene (34.5±6.8 Ma) [16] and that Oryza emerged very recently, by the Middle Miocene period (15–14) [10] . However, beyond these analytical age-estimates, very little is known about the evolutionary history of ehrhartoid grasses, and the rice tribe in particular. The macrofossil record of these groups is virtually absent, with the oldest known macrofossil of the Oryzeae extending back only to the Late Miocene [20] , [21] . Prasad et al . [22] described microscopic silica bodies (phytoliths) of grasses in dinosaur coprolites from the Late Cretaceous period (67–65 Ma) of India, some of which showed affinity to the Ehrhartoideae ( Matleylites indicum ) but could not be clearly assigned to this subfamily based on available data. The coprolites studied by Prasad et al . were recovered from the Maastrichtian (67–65 Ma) Lameta Formation, which consists of alluvial to limnic sediments associated with the Deccan Volcanics (infra- and inter-trappean) of Central India. These deposits are known for their wealth of fossils, including dinosaur bones, coprolites, egg–shell fragments, remains of turtles, frogs, fishes and mammals, as well as macro- and micro-floral remains [23] , [24] , [25] . Continued sampling [22] , [26] , [27] both from Lameta Formation sediments and associated titanosaurid sauropod coprolites from Pisdura (east and south sections) and sediments of the Lameta Formation at Dhamni, Piraya and Polgaon has yielded grass pollen and additional leaf cuticle with embedded grass silica short cell (GSSC) phytoliths similar to those found in oryzoid grasses (often referred to as 'oryzoid' silica bodies [28] ). Here we report on these newly recovered fossil cuticles and associated phytoliths (referred to as morphotypes Changii indicum and Tateokai deccana ) and use them to suggest a different scenario and timing for the emergence and diversification of the rice tribe than what is widely assumed among evolutionary biologists. We first infer a phylogenetic tree for the Poaceae based on molecular and morphological data, which allows us to deduce the placement of the new fossils in the context of 56 extant grass species. Divergence times for Poaceae lineages are then estimated using seven previously published fossils and our new fossils, and this framework is employed to investigate the evolutionary history of seven leaf epidermis and phytolith morphology characters. These characters were also scored for 14 taxa formerly used in phylogenetic analysis of the Ehrhartoideae [10] . Our analysis reveals that Changii indicum and Tateokai deccana most likely were members of the Oryzeae, and that diversification of the rice tribe began before the end of the Cretaceous. Systematic palaeontology Fossil phytolith morphotype . Changii indicum ( Fig. 1a ). 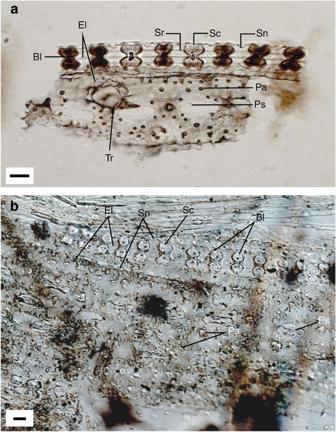Figure 1: Fossil cuticle with phytoliths. (a)Changii indicum, (b)Tateokai deccana. Scale bar,10 μm. Bl=bilobate; El=epidermal long cells; Sn=sinuate margin; Sc=scooped; Sr=silicified ribbed thickening; Pa=papillae; Ps=papillae on subsidiary cells; Tr=trichome. Figure 1: Fossil cuticle with phytoliths. ( a ) Changii indicum , ( b ) Tateokai deccana . Scale bar,10 μm. Bl=bilobate; El=epidermal long cells; Sn=sinuate margin; Sc=scooped; Sr=silicified ribbed thickening; Pa=papillae; Ps=papillae on subsidiary cells; Tr=trichome. Full size image ICPN name . Vertical bilobate/cross with pointed lobes epidermal short cell+rectangular sinuate multi-papillate epidermal long cells+papillate subsidiary cells. Etymology . Genus named in honour of Te-Tzu Chang, who has done pioneering work on the biosystematics, evolution and biogeography of rice, including theories regarding a Gondwana origin of rice: species referring to the country India. Holotype . One piece of cuticle, BSIP 13160 (Q-14-3). Locality and horizon . Coprolites from Red clays, Lameta Formation; Pisdura East and Pisdura South ( Fig. 2 ). 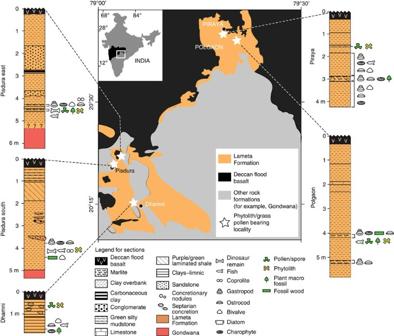Figure 2: Map and stratigraphy of localities. The localities have yielded grass epidermis and phytoliths in coprolites (Pisdura East and South) and in sediment (Dhamni, Piraya and Polgaon) of the Late Cretaceous (Maastrichtian) Lameta Formation in Central India26. The Polgaon and Pisdura East sections have also produced grass pollen. Figure 2: Map and stratigraphy of localities. The localities have yielded grass epidermis and phytoliths in coprolites (Pisdura East and South) and in sediment (Dhamni, Piraya and Polgaon) of the Late Cretaceous (Maastrichtian) Lameta Formation in Central India [26] . The Polgaon and Pisdura East sections have also produced grass pollen. Full size image Other referred specimens: BSIP 13152 (H-28-1), BSIP 13152 (H-27), BSIP 13153 (T-14), BSIP 3161 (Q-29-1). Generic Diagnosis . Costal area (overlying vein) of grass leaf consisting of eight closely spaced, bilobate GSSC arranged in a row on sinuate, distinctly silicified, ribbed, thickened, epidermal long cells. The remaining epidermal long cells have numerous thin-walled, more or less evenly distributed, simple conical papillae, some of which show bifurcation at the base. The subsidiary cells are distinctly quadri-papillate. The GSSC are highly regular in their morphology with well-developed shanks and lobes. The bilobates have markedly scooped ends and are oriented with their long axis at right angles to the papillate epidermal long cells (vertically), showing the characteristic 'oryzoid' pattern. Specific diagnosis . As for genus. Fossil phytolith morphotype . Tateokai deccana ( Fig. 1b ) ICPN name . Vertical bilobate with scooped-end epidermal short cell+rectangular sinuate multi-papillate epidermal long cells. Etymology . Genus named in honour of Tuguo Tateoka, who has done extensive work on the morphology, anatomy, and systematics of the rice tribe and relatives; species referring to the Deccan intertrappean beds. Holotype . One piece of epidermal tissue, SCPGNU 1 (C-48-3). Locality and horizon . Septeria concretions in clays Lameta Formation, Dhamni ( Fig. 2 ). Generic Diagnosis . Costal area of grass leaf consisting of four rows of 14–17 closely spaced bilobate GSSC arranged on rows of epidermal long cells. Remaining epidermal long cells have numerous, thin-walled, densely distributed, simple and bifurcated, long papillae. The subsidiary cells have 2–4 papillae. The GSSC are highly regular in their morphology with well-developed shanks and lobes. The bilobates have deeply scooped ends and are oriented with their long axis at right angles to the papillate epidermal long cells (oryzoid pattern). Specific diagnosis . As for genus. Additional fossil phytolith morphotypes Apart from these more complete specimens, a variety of phytolith morphotypes with more or less clear affinity to Ehrhartoideae based on the distribution of anatomical traits across Poaceae in our analysis (see below), have been found in addition to those reported in Prasad et al . (2005). These include an isolated row of vertical scooped end bilobate/cross and attached papillate epidermal long cells (BSIP 1380, L-48‐2), isolated scooped end bilobate (GSSC) referred as Matleyites indicum (BSIP 13162, K-2; BSIP 13162, K-56‐4; BSIP 13153, T-19‐2)], and one specimen of papillate long epidermis along with two associated keystone bulliform morphotypes characteristic of Bambusoideae and Ehrhartoideae clades (BSIP 13153, P-26‐3). Character analysis of modern reference samples The Joinvillaceae, one of the putative sister groups of grasses, share with the Poaceae the unique division into long cells and short cells of the epidermis, with at least some short cells containing silica [13] ; the other closely related taxa (for example, Ecdeiocoleaceae and Flagellariaceae) lack this arrangement or any well-defined phytoliths [29] . Silica short cells with distinctive bilobate or cross shape, organized in costal rows, such as those found in Changii indicum and Tateokai deccana are exclusive to the grass family [29] (C.A.E.S., unpublished data), firmly establishing the affinity of the fossils to the Poaceae. Although many of the grasses included in the overall Poaceae dataset have been previously investigated [22] , some of the character state scores differ in the current study. These changes are a result of further research, and slightly different and more rigorous definition of characters and character states. For example, the genera Lithachne , Olyra and Pariana (all commonly placed in the Olyreae) are reported in the literature as having 'oryzoid' bilobates, meaning that they are oriented with their long axis perpendicular to the epidermal long cells [28] , and they were scored as such in Prasad et al . [22] as part of the conservative, inclusive approach to character state assignment taken in that paper. However, on careful inspection of phytoliths from these taxa, we find that their costal short cells are very different from the scooped bilobates of the Oryzeae ( Fig. 3 ). They are most commonly cross-shaped and characterized by a 'top', consisting of a more or less flat plate with square lobes at the corners, with the 'base' demarcated by four large bumps or nodules at the lobes ( Fig. 3a,b ). Piperno [30] , [31] , [32] recognized this distinct shape as 'cross variant 3 and 8.' Similarly, although Pseudosasa is not included in the phylogenetic analysis, it can be noted that its bilobates do not have well-developed shanks of typical Oryzeae bilobates and many have an extra lobe along the shank, making them more similar to polylobate or crenate forms ( Fig. 3d ). 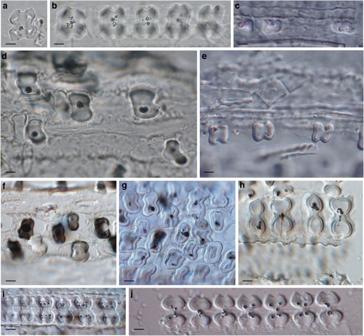Figure 3: Examples of samples from modern reference collection material used in this study. (a,b) Cross variant 3 and 8 with a nodule at each lobe (Lithachne pauciflora); single bilobate (a), in a row (b). (c) Row of horizontally oriented oblong bilobates (Ehrhartasp.). (d) Row of bilobates grading into polylobate or crenate short cells (Pseudosasa usawai). (e) Row of horizontal bilobates (Potamophilasp.). (f,g) Vertical bilobates with rounded ends arranged randomly in the leaf tissue;Zizaniopsissp. (f),Rhynchoryzasp. (g). (h) Row of vertical bilobates with rounded to slightly concave ends (Zizaniasp). (i,j) Row of vertical bilobates-crosses with deeply concave (scooped) ends;Leersia hexandra(i),Oryza sativa(j). Scale bar, 5 μm. Figure 3: Examples of samples from modern reference collection material used in this study. ( a , b ) Cross variant 3 and 8 with a nodule at each lobe ( Lithachne pauciflora ); single bilobate ( a ), in a row ( b ). ( c ) Row of horizontally oriented oblong bilobates ( Ehrharta sp.). ( d ) Row of bilobates grading into polylobate or crenate short cells ( Pseudosasa usawai ). ( e ) Row of horizontal bilobates ( Potamophila sp.). ( f , g ) Vertical bilobates with rounded ends arranged randomly in the leaf tissue; Zizaniopsis sp. ( f ), Rhynchoryza sp. ( g ). ( h ) Row of vertical bilobates with rounded to slightly concave ends ( Zizania sp). ( i,j ) Row of vertical bilobates-crosses with deeply concave (scooped) ends; Leersia hexandra ( i ), Oryza sativa ( j ). Scale bar, 5 μm. Full size image Fossil placement and estimation of ancestral character states The phylogenetic analysis showed that the fossils form a clade with in the Oryzeae (posterior probability=0.8) and more inclusively within the Ehrhartoideae (posterior probability=0.88) and display a combination of vertical bilobates in the costal row (character 2; Table 1 ) with scooped shape (character 3), papillate long cells (character 5), and papilla on the subsidiary cells of the stomata (character 6) ( Fig. 4 ). Bayesian estimation of ancestral character states for characters 2 and 5 indicates that these character states evolved in the Oryzeae and, hence, are derived with respect to the Ehrhartoideae. An anatomical survey of many of the species and genera used in phylogenetic analysis of Oryzeae [10] confirms the presence of these traits in all studied Oryzeae genera ( Supplementary Table S1 ). Papilla on long cells appear to have evolved independently in the Bambusoideae as well as in the Puelioideae and certain PACMAD taxa (represented by Distichlis , Amphipogon and Micraira ) ( Fig. 4 ). Our analysis and survey of Oryzeae taxa further suggest that vertical bilobates with scooped shape (character 3) are unique to taxa nested in the Oryzeae ( Supplementary Table S1 ). In addition, papillate stomatal subsidiary cells (character 6), seem to have evolved in the closely related genera ( Oryza and Leersia ) within the Oryzeae tribe, as well as in certain bambusoid taxa ( Chusquea and Olyreae, represented by Lithachne and Olyra ) ( Fig. 4 ; Supplementary Table S1 ). Remaining characters (1, 4 and 7) are either highly homoplastic (character 1) or have too much missing data (4 and 7) to be informative with respect to character evolution and phylogenetic placement of the fossil taxa. Table 1 Morphological characters and character states. 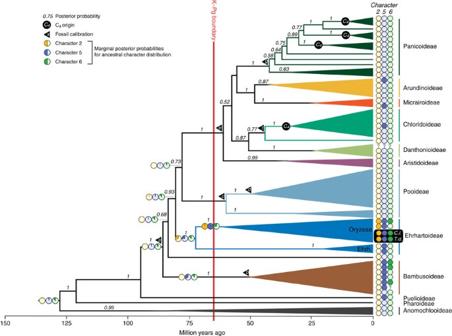Figure 4: Character state evolution of three of the seven leaf epidermal and phytolith characters across Poaceae. Poaceae timetree estimated using BEAST version 1.6.1. Placement of the fossils are based on MrBayes phylogenetic analysis based on molecular and morphological data (Supplementary Fig. S1). Pie charts indicating marginal posterior probability distributions (dark shades=presence; light shades=absence of trait). Preferred placement of grass fossils emphasized by black box. Cretaceous–Paleogene (K–Pg) boundary marked with red vertical line.C.i.=Changii indicum;T.d.=Tateokai deccana. Characters: 2=vertical bilobates in costal row; 5=papilla on epidermal long cells; 6=papilla on subsidiaries of stomata. Full size table Figure 4: Character state evolution of three of the seven leaf epidermal and phytolith characters across Poaceae. Poaceae timetree estimated using BEAST version 1.6.1. Placement of the fossils are based on MrBayes phylogenetic analysis based on molecular and morphological data ( Supplementary Fig. S1 ). Pie charts indicating marginal posterior probability distributions (dark shades=presence; light shades=absence of trait). Preferred placement of grass fossils emphasized by black box. Cretaceous–Paleogene (K–Pg) boundary marked with red vertical line. C.i. = Changii indicum ; T.d. = Tateokai deccana . Characters: 2=vertical bilobates in costal row; 5=papilla on epidermal long cells; 6=papilla on subsidiaries of stomata. Full size image Dating analysis Because of the relatively low branch support (0.8) for the preferred placement of the fossils as part of Oryzeae, we considered three alternative placements of the fossils for the dating analysis: at the base of Ehrhartoideae (H 1 ), at the base of a clade consisting of PACMAD and Pooideae (H 2 ), and at the base of the (PACMAD, Ehrhartoideae) clade (H 3 ) ( Supplementary Fig. S1 ). Dating using BEAST showed that inclusion of the new fossils affects dating of all nodes regardless of where they are placed (preferred placement, H 1 –H 3 ) ( Table 2 ; Supplementary Fig. S2 ). However, the effect is greatest when the fossils are placed in Oryzeae (preferred placement) and is larger both in absolute terms (millions of years) and proportionally for deeper nodes. For example, for the (Bambusoideae, PACMAD) clade, the most conservative hypothesis for the placement of the fossils, H 3 , results in a >6% older date (76 Ma as opposed to 72 Ma without the new fossils), whereas the preferred placement results in a 20% difference (86 Ma). The corresponding difference for the much younger clade of C 4 grasses within the Paniceae X=9 group is a <6% difference (19 Ma instead of 18 Ma) for H 3 and 13% (20 Ma) for the preferred placement of the fossils. The largest effect is on the date for the origin of the clade that includes Oryzeae and the fossils under the preferred placement, with a difference in age of 124% (63 Ma instead of 28 Ma). The preferred placement produces an age for the root of Poaceae of 128 Ma, 20% older than when the new fossils are excluded; ages for H 1 –H 3 range from 115 to 121 Ma. Table 2 Dating analysis, showing that divergence times differ substantially when the new fossils are included ( Supplementary Fig. S9 ). Full size table Whereas some leaf anatomical and phytolith characters analysed in this study are less phylogenetically informative because they are either highly homoplastic (arrangement of GSSCs) or too much data are currently missing (for example, silicification of cells that bear GSSCs), several characters, when carefully defined, are clearly useful for placing well-preserved fossils in the phylogeny. The Bayessian estimation of ancestral character states across Poaceae, supplemented by our survey of grasses within the Ehrhartoideae, indicate that, among extant grasses, vertically oriented bilobate GSSCs with scooped shape are found exclusively in members of tribe Oryzeae of the Ehrhartoideae subfamily. Previous workers have lumped vertically oriented ('oryzoid') silica bodies produced by several grass genera, for example, Eriachne , Psuedosasa and the Olyreae (for example, Pariana , Lithachne and Olyra ), with those typical of Oryzeae [28] , [33] . As a result, these types of GSSCs have been considered only moderately useful from a phylogenetic perspective [34] . In contrast, through the more in-depth study of this character, we found that the bilobate and cross-shaped silica bodies in grasses outside the rice tribe are very different in three-dimensional morphology from the vertical bilobates that signify members of Oryzeae ( Fig. 3 ), and therefore not directly comparable. The substantial phylogenetic distance separating the taxa that produce different types of vertical silica bodies also supports the hypothesis that this aspect of GSSC morphology is a result of convergence, not common ancestry. Papillate epidermal long cells and papillate stomatal subsidiaries also appear to be diagnostic of certain members of the Oryzeae, although these traits are also found in a few taxa outside this group ( Fig. 4 ; Supplementary Table S1 ). The distribution of character states across Poaceae and the combination of character states in the grass fossils indicate that both Changii indicum and Tateokai deccana belong in the Oryzeae, although the reconstruction yields relatively low support. Alternative placements suggested by the phylogenetic analysis nevertheless make both fossils derived with respect to modern subclades such as Bambusoideae. This placement of the Late Cretaceous fossils has radical implications for the amount of diversification that had taken place within the Poaceae at the close of the Mesozoic era. In the phylogeny used herein, it can be inferred that, by 65 Ma (K–Pg boundary), the Ehrhartoideae had split from the Pooideae+PACMAD lineage [18] , or else from the other clades within the BEP [13] , [16] , [17] . In addition, the Oryzeae must have split from the Ehrharteae within the Ehrhartoideae. In our dating analysis, placing the fossils as part of the Oryzeae results, not surprisingly, in extremely old dates for the Ehrhartoideae and Oryzeae (72 Ma and 63 Ma, respectively). These dates contrast sharply with the divergence times yielded when only the seven published fossils are used to calibrate the tree (49 Ma and 28 Ma, respectively), and with dates proposed previously based on molecular clock work, namely a late Middle or even Late Eocene (40–35 Ma) origin of the Ehrhartoideae, and a Late Eocene–Early Oligocene ( ∼ 25 Ma) origin of the Oryzeae [16] , [17] , [18] . Similarly, the preferred placement of the fossils leads to dates for the origin of the Pooideae and the PACMAD clade that are >20 myr older than published estimates of 39–44 Ma and 38–44 Ma, respectively [16] , [17] , [18] . These differences are in large part due to the inclusion of the fossils described in this paper, but also to some extent a result of consideration of recently published fossils from Patagonia, Argentina ( Supplementary Table S2 ). In addition, our use of certain fossil calibration points differs from previous studies. For example, we use the Chusquea -like fossils described from the Late Eocene of North America as a calibration point for the Bambusoideae, whereas Vicentini et al . [16] used it to calibrate the BEP–PACMAD split. Note that we did not include the fossils described by Prasad et al . [22] because of the uncertainty in the taxonomic affinities of these fossils. Two sets of dates inferred from our dating analysis are of particular interest. First, under the preferred position of the fossils, we place the oldest origin of C 4 grasses, in the Chloridoideae, in the latest Eocene as opposed to the Early Oligocene (<32 Ma), as deduced in former studies [16] , [17] , [18] , [35] . This early timing is consistent with the discovery of C 4 grass pollen from the earliest Oligocene of Spain [36] , and indicates that some C 4 grasses evolved under the high (>1,000 p.p.m.) atmospheric CO 2 of the Eocene and earliest Oligocene. It has been generally assumed that the C 4 photosynthetic pathway, which today confers an advantage to plants in climates characterized by high temperatures, aridity, summer precipitation, as well as at low pCO 2 (ref. 37 ) could have evolved only after CO 2 levels had dropped well below 1,000 p.p.m. after the earliest Oligocene (<32 Ma) [16] , [18] , [35] , [38] . The possible appearance of grasses with C 4 photosynthesis before this time means that a mechanism other than low CO 2 must be invoked for the evolution of this trait, for example, aridity combined with the relatively elevated temperatures in the Late Eocene [36] , [39] . Second, our analyses yield markedly older dates for the origin of the grass family than previous work—regardless of the placement of the new fossils. The estimated age of the Poaceae inferred herein range from 107 Ma (new fossils excluded) to 129 Ma (preferred placement of fossils), compared with published ages of ∼ 70–95 Ma (refs 16 , 17 , 18 , 40 ). These new, very old dates for the Poaceae would likely also result in more ancient ages for the monocotyledons and angiosperms as a whole. Molecular clock analyses constrained by the known fossil record of angiosperms have typically provided ages of, respectively, 120–130 Ma and 140–190 Ma, for these groups [41] , [42] , [43] . However, several recent molecularly based dating analyses of land plants point to significantly older dates, with monocotyledons emerging in the Late Jurassic period (161–145 Ma) [44] and angiosperms in the Late Triassic period (235–202 Ma) [44] , [45] . Our estimated age for the Poaceae is more consistent with these latter analyses. To reconcile these wildly disparate outcomes for the ages of grasses and flowering plants, it may be necessary to re-examine presently employed rate models in molecular clock dating and ways of implementing fossil calibration points [44] , [45] , as well as to expand and refine our knowledge of Late Cretaceous grasses through paleontological fieldwork and phylogenetic analysis. Our study, therefore, reinforces the importance of the growing record of fossil phytoliths [22] , [46] , [47] for shedding light on the hitherto obscure evolutionary history of grasses. Grasses are today notoriously widespread and attempts at reconstructing the ancestral area of the group using current biogeographic ranges have remained inconclusive, although a Gondwanan origin is widely assumed [17] , [48] . The fossils described herein, representing a very early stage in the history of the Poaceae, combined with the recalibrated grass phylogeny have the potential of shedding some light on this question. Our recalibration suggests that the grass clade had diversified substantially by the K–Pg transition ( Fig. 4 ); the question is, did this diversification occur on the Indian subcontinent or elsewhere? Because India was biogeographically isolated during the time when the Lameta Formation was deposited [49] , one possibility is that the Poaceae underwent most of its initial taxonomic radiation in India during this isolation. Dispersal of the major grass lineages would have taken place only after India made contact with the South Asian margin in the Early Eocene period ( ∼ 55 Ma) [49] , [50] . An alternative scenario that is more concordant with our new, ancient dates for major splits within Poaceae is one in which diversification and dispersal of grass lineages among at least some Gondwanan continents preceded the loss of a land bridge between India and the rest of Gondwana at ∼ 80 Ma (refs 51 , 52 ). This hypothesis would also agree better with a recent phylogenetic effort to reconstruct Poaceae biogeographic history that proposes an African origin for both BEP+PACMAD and BEP [17] , because it would imply that these lineage divergences occurred while Africa and India were still in contact. Such a biogeographic scenario remains to be tested in the fossil record; so far, sediment samples from Africa (Madagascar) of Late Cretaceous age have not yielded any (grass or other) phytoliths (Strömberg, unpublished data). Extraction process Coprolites collected from the Pisdura area ( Fig. 2 ) were processed by V.P. After thorough cleaning of the surface, ∼ 2 g of material was taken from the inside of the coprolites. The samples were treated with 40% HCl to remove carbonates, 40% H 2 O 2 to oxidize excess organic material and 5% sodium hexa-meta-phosphate to remove clays. The Lameta sediment samples from Pisdura, Piraya and Dhamni locality were collected and processed using similar methods by B.S. The residue was mounted in Canada Balsam for viewing under a light microscope at ×400 and ×630 magnification and immersion oil. Description of fossil phytolith morphotypes Fossil cuticles have been given unique names for reference. Protocols for phytolith description and assigning nomenclature are the same as carried out in a previous study [22] . Slides with fossil phytoliths are housed in the repository of the Birbal Sahni institute for palaeobotany (BSIP), Lucknow, and Postgraduate Department of Geology, Rashtrasant Tukadoji Maharaj Nagpur University, Nagpur, India. For each specimen, the number (for example, BSIP 13160) refers to the slide; this is followed by England Finder coordinates. Modern reference samples Leaves of fourteen modern Ehrhartoideae species from nine genera were sampled in the Laboratory of Systematic and Evolutionary Botany, Chinese Academy of Sciences, Beijing, China; Phyllostachys material was collected at the National Botanical Research Institute. In addition, phytoliths extracted from 46 grass taxa ( Fig. 4 ; Strömberg, unpublished data) were studied and complemented by information from the literature [28] , [32] , [33] . Because the sister groups of the Poaceae (Joinvillaceae, Ecdeiocoleaceae and Flagellariaceae) lack well-defined GSSCs [29] (C.A.E.S., unpublished data), we did not include these in the modern reference set (see Discussion ). The material was scored for seven epidermal/phytolith characters ( Table 1 ). Character states were assigned using what appear to be natural breaks in variation; future studies will attempt to refine this scheme through quantitative, statistically based subdivision of character states which was not possible in this study. Phylogenetic analysis A phylogeny for the Poaceae was estimated through Bayesian inference using MrBayes v3.1.2 (ref. 53 ) with a combination of plastid molecular data ( rbcL and ndhF ) from Christin et al . [18] ( Supplementary Table S3 ) and a new morphological dataset. The Christin et al . dataset was reduced to 56 taxa for which anatomical data were available, with Anomochlooideae ( Anomochloa , Streptochaeta ) used as the outgroup. The rbcl and ndhF genes (3,463 bp) were partitioned and modelled using the GTR+I+ Γ model of nucleotide substitution (all parameters were unlinked) and combined with a morphological dataset containing seven characters ( Supplementary Table S1 ). The morphological data used the MK model (Markov k model [54] ), and this dataset included the 56 taxa with molecular data as well as the two new fossil taxa (with no molecular data). As none of the morphological characters were constant, we used the commands 'coding=variable' and 'rates=gamma' in MrBayes. Four separate analyses were run; each initiated with a different random starting seed. The analyses used four heated Markov chains (using default heating values) that were run for 50 million generations with sampling intervals of 10,000 steps. Convergence was assessed by inspecting the cumulative posterior probabilities of clades and by comparing the posterior probability values across multiple runs using the online program 'Are we there yet?' [55] ( Supplementary Figs S3–S6 ). Posterior probability values were obtained by summarizing the posterior distribution of trees (post burn-in) with a 50% majority-rule consensus tree ( Supplementary Fig. S1 ). Ancestral character state estimation Ancestral character states were estimated using Bayesian inference in BayesTraits v1.0 (refs 56 , 57 ). Advantages of the Bayesian approach are that it uses reversible-jump Markov chain Monte Carlo to average over all k -state models of character evolution and accommodates uncertainty in the phylogeny and the rate parameters of the models [58] . Bayesian inference of ancestral character states was conducted using all post-burn-in trees from the posterior distribution of phylogenies obtained from the MrBayes analysis of the combined molecular and morphological data. Utilizing this posterior distribution of trees allowed us to include the new fossil taxa in the ancestral character state estimation procedure. The BayesTraits analyses were run for 10 million generations, sampling at intervals of 10,000 steps after a burn-in period of 100,000 steps. The rate deviation parameter was set, so that the resulting acceptance rates fell between 0.2 and 0.4 (generally 0.26–0.30). The average of the resulting posterior probability distributions was used to produce final estimates of the probabilities for ancestral state estimates ( Supplementary Table S4 ). We repeated these analyses with a revised posterior distribution of trees that excluded the new fossil taxa to examine the impact of these taxa on ancestral state estimations. Dating analysis We estimated divergence times for the Poaceae using BEAST v1.6.1 (ref. 59 ). These analyses utilized the same molecular genetic data and partitioning strategy used in the MrBayes analysis (56 taxa, 3,463 characters, 2 gene partitions). We inferred divergence times by assigning seven fossil calibrations to the tree either in combination with or separately from the new fossil taxa described here ( Table 2 ; Supplementary Table S2 ; Supplementary Figs S7 and S8 ). Uncertainties in the fossil calibrations were incorporated into the divergence dating analysis using lognormal prior distributions with soft bounds (no zero offset). We parameterized the log(mean) and log(standard deviation) values of the lognormal distributions using ParameterSolver v.2.3 ( https://biostatistics.mdanderson.org/SoftwareDownload/ ) so that the upper and lower absolute dates represented the 2.5 and 97.5% quantiles of the distribution. We also examined the impact of each of the seven fossil calibrations by systematically removing each one from the analysis and evaluating the change in the posterior distributions for divergence times ( Supplementary Fig. S9 ). For all analyses, substitution rate variation among lineages was modelled using an uncorrelated lognormal distribution, and we ran the analyses under the birth–death branching prior. Monophyly was not enforced for any nodes. The MCMC analyses were run for 20 million generations, logged every 1,000 steps, and the divergence times for nodes of interest were sampled at the same frequency. We used Tracer v 1.5 to determine convergence, measure the effective sample size of each parameter, and calculate the mean and 95% highest posterior density (HDP) interval for divergence times [60] . How to cite this article: Prasad, V. et al . Late Cretaceous origin of the rice tribe provides evidence for early diversification in Poaceae. Nat. Commun. 2:480 doi: 10.1038/ncomms1482 (2011).